Dissecting the role of H3K64me3 in mouse pericentromeric heterochromatin To ensure genome stability, pericentromeric regions are compacted in a dense heterochromatic structure through a combination of specific ‘epigenetic’ factors and modifications. A cascadal pathway is responsible for establishing pericentromeric chromatin involving chromatin modifiers and ‘readers’, such as H3K9 histone methyltransferases (Suv)39h and heterochromatin protein 1. Here we define how H3K64me3 on the lateral surface of the histone octamer integrates within the heterochromatinization cascade. Our data suggest that enrichment of H3K64me3 at pericentromeric chromatin foci is dependent on H3K9me3 but independent of a number of central factors such as heterochromatin protein 1, DNA methyltransferases and Suv4-20h histone methyltransferases. Our results support a model in which pericentromeric heterochromatin foci are formed along distinct pathways upon H3K9 trimethylation, involving H3K64me3 to potentially stabilize DNA–histone interactions, as well as sequential recruitment of repressive histone tail and DNA modifications. We hence suggest that multiple mechanisms ensure heterochromatin integrity at pericentromeres, with H3K64me3 as an important factor. Epigenetic regulation of genome function is a fundamental principle of cellular activity. Chromatin, the totality of genomic DNA and associated histone and non-histone proteins, forms the platform by which epigenetic information translates into genomic activity. Two principal types of chromatin are present within the nucleus: accessible ‘euchromatin’ and more densely packed ‘heterochromatin’ [1] , [2] . Heterochromatin exists as ‘facultative heterochromatin’, which is of a more temporary nature and forms, for example, at developmentally regulated gene loci under the influence of cellular signals. In contrast, ‘constitutive heterochromatin’ remains stably condensed and is preferentially formed at chromosomal regions with high densities of repetitive DNA elements [2] . A total of 44% of the mouse genome accounts for such repetitive elements, classed into short interspersed repeats and tandem repeats, the latter of which constitute the pericentromeric, centromeric and telomeric regions [3] . Silencing of DNA repeats through constitutive heterochromatinization is thought to be crucial for maintaining genome stability. This heterochromatinization minimizes recombination events initiated by interspersed repeats and ensures correct chromosomal structuring and unperturbed mitotic chromosome segregation at tandem repeat regions [2] , [4] , [5] , [6] . In the mouse, pericentromeric heterochromatin contains a basic, AT-rich, 234pb-long DNA repeat termed γ-satellite or major satellite [7] , [8] . In interphase cells, major satellites from individual chromosomes cluster to form distinct entities or ‘chromocenters’, which can be easily detected as DAPI (4',6-diamidino-2-phenylindole)-rich foci [5] , [9] . Specific covalent modifications are characteristically associated with pericentromeric heterochromatin. These are the histone lysine modifications H3K9me3, H4K20me3, H3K27me1, the more recently characterized H3K64me3, as well as CpG DNA methylation [3] , [10] , [11] . These markers are important for proper heterochromatinization, and several studies suggest that their placement follows a hierarchical sequence of events [12] , [13] , [14] , [15] . One of the most upstream events in the cascade of pericentromeric heterochromatin formation appears to be the targeted trimethylation of H3K9, catalysed through the activity of suppressor of variegation (Suv) 39h1 and Suv39h2 enzymes that convert H3K9me1 into H3K9me3 [16] , [17] , [18] . The mechanism by which Suv39h enzymes are specifically recruited to pericentromeric regions in the mammalian genome is unclear. Although it is well established that in Schizosaccharomyces pombe this recruitment involves an RNA-mediated interference (RNAi)-dependent mechanism, initiated by transcriptional activity on pericentromeric repeats, no such RNAi-based mechanism has been found in mammalian cells [2] , [11] , [19] , [20] . In mammals, enrichment of H3K9me3 results in the recruitment of chromodomain-containing proteins, such as heterochromatin protein 1 (HP1), in particular the HP1α and ß isoforms. HP1 binding promotes further heterochromatinization by directing several enzymatic activities to chromatin [5] , [12] , [13] . First, HP1 associates with Suv4-20h1 and Suv4-20h2 enzymes, both catalysing the trimethylation of H4K20 and chromatin compaction [15] , [21] . Furthermore, it acts as a binding platform for the DNA methyltransferase Dnmt3b, resulting in the enrichment of methyl-CpG at these regions [14] . HP1 also associates with Suv39h and thereby further enhances H3K9me3 levels, creating a positive feedback loop for heterochromatin stability and spreading [5] , [22] . Finally, the formation of constitutive heterochromatin at pericentromeric repeats is stabilized through binding of the methyl-CpG-binding protein MeCP2 and associated histone deacetylase and additional histone methyltransferase activities [23] , [24] , [25] . We have previously identified trimethylation of H3K64 as a novel constituent of pericentromeric heterochromatin [10] , to which it colocalizes together with markers of repressive chromatin, such as H3K9me3 and DNA methylation. H3K64 resides in the globular domain of H3 and is located at the lateral surface of the histone octamer, close to the DNA. H3K64me3 is ubiquitous in human and mouse cell lines and tissues. During mammalian development, H3K64me3 is dynamically remodelled in the context of genomic reprogramming despite its location. We have proposed that H3K64me3 could help create a repressive chromatin state. Indeed, it was shown that H3K64me3 is depleted from active promoter regions and sites of RNA PolII activity but it is enriched at constitutively silenced, repetitive DNA elements, including pericentromeric heterochromatin. To dissect the role of H3K64me3 in the formation, maintenance and function of pericentromeric heterochromatin, in this study we set out to investigate how trimethylation of H3K64 integrates in vivo within the well-characterized pathway of heterochromatinization at pericentromeric repeats. We made use of a number of mutant cell lines deficient for the key factors of this pathway and systematically explored the dependency of H3K64me3 targeting and maintenance on these factors. Our results suggest that enrichment of H3K64me3 at pericentromeric heterochromatin foci occurs in a manner that is dependent on H3K9me3 but independent of DNA methylation, H4K20me3 or HP1. Our findings strongly argue for a role of H3K64me3 as a novel key component of heterochromatin integrity at pericentromeric sites. Pericentromeric H3K64me3 foci are independent of DNA methylation Two important features of H3K64me3 are the fact that H3K64me3—a modified site localized to the nucleosomal core—is substantially remodelled during genome-wide epigenetic reprogramming following fertilization in mouse zygotes [26] , [27] and that it shows local correlation with DNA methylation in cell culture [10] . As levels of DNA methylation are known to change drastically during epigenetic reprogramming periods [28] , [29] , [30] , we first asked whether H3K64me3 correlates with DNA methylation changes globally in vivo . For this, we performed double immunostaining with anti-H3K64me3 and anti-5-methyl-cytosine (5mC) antibodies in mouse zygotes. The latter contain CpG-methylated maternal and unmethylated paternal pronuclei [31] . As shown in Fig. 1a , H3K64me3 is not detectable in unmethylated paternal chromatin and significantly colocalizes with 5mC in the maternal chromatin ( Fig. 1a ; 68.2% of H3K64me3 signal colocalized with 5mC). Hence, local correlation of H3K64me3 and DNA methylation at constitutive heterochromatin is also present in vivo during stages of epigenetic remodelling. 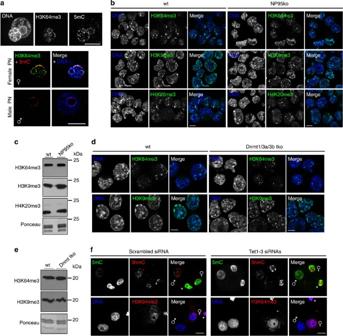Figure 1: Enrichment in pericentromeric foci and global levels of H3K64me3 are independent of global DNA methylation. (a) Mouse zygotes were immunostained with 5mC and H3K64me3 antibodies and analysed under confocal microscopy. The paternal pronucleus is largely devoid of H3K64me3 and 5mC. Shown are full projections of Z-sections (upper panels) or one merged single section (lower panels). Male and female pronuclei (PN) are indicated. Scale bar, 10 μm. Quantification revealed that 68.2% of DNA-methylated regions are stained by H3K64me3. (Standard deviation=11%,n=14). (b) Immunofluorescence (IF) analysis of wild-type (wt, left panels) and NP95−/− (right panels) ES cells using antibodies against H3K64me3, H3K9me3 and H4K20me3. DNA was counterstained with DAPI. NP95 mutant cells show pericentromeric localization of H3K64me3, H3K9me3 and H4K20me3 comparable with wt. Scale bar, 10 μm. (c) Immunoblot analysis of native histones extracted from wt and NP95−/− cells using antibodies against H3K64me3, H3K9me3 and H4K20me3. Loading was controlled by Ponceau staining. Note that levels of all three H3 methylations are comparable in ko and wt extracts. (d) IF analysis of wt (left panels) and Dnmt1/3a/3b triple ko (right panels) ES cells indicates similar patterns of H3K64me3 and H3K9me3 at DAPI-intense foci corresponding to pericentromeric heterochromatin (PH). Scale bar, 10 μm. (e) Native histone extracts of wt and Dnmt1/3a/3b triple ko ES cells show comparable levels of H3K64me3 and H3K9me3 in immunoblot analysis. Loading was controlled by Ponceau staining. (f) Zygotes treated with scrambled control siRNA (left panels) and Tet 1/2/3 siRNAs (right panels) were analysed by IF staining for 5mC, 5hmC and H3K64me3 levels. DNA was counterstained with DAPI. Tet 1/2/3 siRNA-treated zygotes show distinct increase in 5mC levels at the paternal pronucleus, which, however, does not coincide with an increase in H3K64me3. Asterix indicates the polar body. Scale bar, 20 μm. Figure 1: Enrichment in pericentromeric foci and global levels of H3K64me3 are independent of global DNA methylation. ( a ) Mouse zygotes were immunostained with 5mC and H3K64me3 antibodies and analysed under confocal microscopy. The paternal pronucleus is largely devoid of H3K64me3 and 5mC. Shown are full projections of Z-sections (upper panels) or one merged single section (lower panels). Male and female pronuclei (PN) are indicated. Scale bar, 10 μm. Quantification revealed that 68.2% of DNA-methylated regions are stained by H3K64me3. (Standard deviation=11%, n =14). ( b ) Immunofluorescence (IF) analysis of wild-type (wt, left panels) and NP95−/− (right panels) ES cells using antibodies against H3K64me3, H3K9me3 and H4K20me3. DNA was counterstained with DAPI. NP95 mutant cells show pericentromeric localization of H3K64me3, H3K9me3 and H4K20me3 comparable with wt. Scale bar, 10 μm. ( c ) Immunoblot analysis of native histones extracted from wt and NP95−/− cells using antibodies against H3K64me3, H3K9me3 and H4K20me3. Loading was controlled by Ponceau staining. Note that levels of all three H3 methylations are comparable in ko and wt extracts. ( d ) IF analysis of wt (left panels) and Dnmt1/3a/3b triple ko (right panels) ES cells indicates similar patterns of H3K64me3 and H3K9me3 at DAPI-intense foci corresponding to pericentromeric heterochromatin (PH). Scale bar, 10 μm. ( e ) Native histone extracts of wt and Dnmt1/3a/3b triple ko ES cells show comparable levels of H3K64me3 and H3K9me3 in immunoblot analysis. Loading was controlled by Ponceau staining. ( f ) Zygotes treated with scrambled control siRNA (left panels) and Tet 1/2/3 siRNAs (right panels) were analysed by IF staining for 5mC, 5hmC and H3K64me3 levels. DNA was counterstained with DAPI. Tet 1/2/3 siRNA-treated zygotes show distinct increase in 5mC levels at the paternal pronucleus, which, however, does not coincide with an increase in H3K64me3. Asterix indicates the polar body. Scale bar, 20 μm. Full size image Prompted by this observation, we next set out to investigate whether maintenance and/or localization of H3K64me3 to pericentromeric heterochromatin foci is dependent on DNA methylation. To address this, we first made use of two mutant mouse ES cell lines in which DNA methylation is largely deficient: NP95 knockout (ko) cells (NP95−/−) and Dnmt1/Dnmt3a/Dnmt3b triple ko cells (Dnmt1/3a/3b tko [32] , [33] ). NP95 binds to hemimethylated DNA at the replication fork and interacts with the maintenance DNA methyltransferase Dnmt1, thereby recruiting DNA methylation activity to replicating heterochromatin [34] , [35] . Cells deficient for NP95 show a genome-wide decrease in DNA methylation, with mislocalization of the methyl-CpG-binding protein MeCP2 (Supplementary Fig. S1a), hypomethylation of pericentromeric and centromeric repeats, interspersed repeats and imprinted loci [36] . ES cells genetically deficient for all three known Dnmts show even more pronounced genome-wide hypomethylation, with CpGme retention of only ~0.4% [33] . Figure 1b demonstrates that the pericentromeric foci and overall staining intensity for H3K64me3 are comparable between NP95−/− and wt cells. A similar observation was made for the heterochromatin markers H3K9me3 and H4K20me3 ( Fig. 1b ). In line with this, we detect the usual pericentromeric H3K64me3 foci in Dnmt1/3a/3b tko ES cells ( Fig. 1d ), as well as unaltered H3K9me3 staining pattern ( Fig. 1d ). Our western blot analysis shows no decrease in global H3K64me3 levels on comparing DNA methylation-deficient NP95−/− and Dnmt1/3a/3b tko cells with wt ES cells. Similarly, no decrease was observed for H3K9me3 and H4K20me3 levels ( Fig. 1c,e ; Supplementary Fig. S1c–e [33] ). Note that levels of H3K64me3 are generally constant during the cell cycle ( Supplementary Fig. S1b ). These data demonstrate that presence of the hemi-methylcytosine binder NP95 as well as of three Dnmt proteins is not required for global H3K64me3 levels, nor for its localization at pericentromeric heterochromatin foci. To test whether increased levels of DNA methylation can affect H3K64me3, we employed a second experimental approach by making use of inverse correlating levels of 5-methyl cytosine (5mC) and 5-hydroxymethyl cytosine (5hmC) during early mouse development [37] . Reduction in 5hmC through knockdown of Tet 1/2/3 RNAs results in maintenance of high 5mC levels in the paternal pronucleus ( Fig. 1f [37] ). Such an experimental setup therefore allows to assess whether increased levels of 5mC are sufficient to upregulate H3K64me3 in paternal chromatin. Interestingly, in Tet 1/2/3 RNAi-treated and ICSI-fertilized oocytes, the paternal pronucleus seems to show no enrichment of H3K64me3, which stays restricted to heterochromatic regions in the maternal pronucleus ( Fig. 1f ). Hence, elevation of CpG methylation levels appears to be insufficient for inducing H3K64me3 recruitment at pericentromeric sites. Notably, we cannot exclude the possibility of insufficient de novo H3K64me3 activity at this developmental stage. Taken together, our data strongly suggest that, although locally correlated, the localization of H3K64me3 at pericentromeric heterochromatin foci is independent of DNA methylation levels. Suv4-20 is not required for pericentromeric H3K64me3 foci We next went on to investigate a possible dependency of H3K64me3 on H4K20me3. Two enzymes, Suv4-20h1 and Suv4-20h2, are responsible for catalysing H4K20me3 at the pericentromere. This methylation is unidirectionally dependent on Suv39h in the heterochromatinization pathway [15] , [38] . As expected, Suv4-20h1/h2 double ko mouse embryonic fibroblasts (MEFs) are devoid of H4K20me3 in pericentromeric heterochromatin ( Supplementary Fig. S2a ), whereas the usual pattern of H3K9me3 enrichment at the pericentromere is seen ( Fig. 2a ). In both wt and Suv4-20h1/h2 dko mutant cell lines, the staining pattern for H3K64me3 seems comparable and enriched in heterochromatic foci ( Fig. 2a ). These results were complemented by western blot analysis of mutant and wt control cells, which reveal similar global levels of H3K64me3 in Suv4-20h1/h2 dko mutant and wt cells ( Fig. 2b and Supplementary Fig. S2b ). To conclude, our data demonstrate that the absence of H4K20me3 does not impede on H3K64me3 localization at pericentromeric heterochromatin foci. Furthermore, H3K64me3 at the pericentric heterochromatin, as well as global levels, is not dependent on the Suv4-20 enzymes. 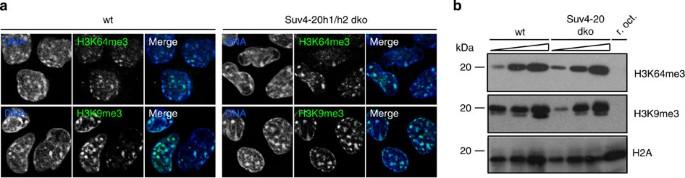Figure 2: Suv4-20 is not required for H3K64me3 localization to PH foci. (a) IF analysis of wt (left panels) and Suv4-20h1/h2 dko (right panels) MEFs using antibodies against H3K64me3 and H3K9me3. DNA was counterstained with DAPI. Suv4-20h1/h2 mutant cells show pericentromeric enrichment of H3K64me3 and H3K9me3 comparable to wt. Scale bar, 10 μm. (b) Immunoblot analysis of native histones extracted from wt and Suv4-20h1/h2 dko MEFs shows no reduction in global H3K64me3 or H3K9me3 levels in dko cells. Increasing amounts of histones were loaded and a control lane was included with recombinant, unmodified octamers (r.oct.) that are not recognized by the different antibodies. Loading was controlled by blotting against H2A. Figure 2: Suv4-20 is not required for H3K64me3 localization to PH foci. ( a ) IF analysis of wt (left panels) and Suv4-20h1/h2 dko (right panels) MEFs using antibodies against H3K64me3 and H3K9me3. DNA was counterstained with DAPI. Suv4-20h1/h2 mutant cells show pericentromeric enrichment of H3K64me3 and H3K9me3 comparable to wt. Scale bar, 10 μm. ( b ) Immunoblot analysis of native histones extracted from wt and Suv4-20h1/h2 dko MEFs shows no reduction in global H3K64me3 or H3K9me3 levels in dko cells. Increasing amounts of histones were loaded and a control lane was included with recombinant, unmodified octamers (r.oct.) that are not recognized by the different antibodies. Loading was controlled by blotting against H2A. Full size image H3K64me3 is enriched at pericentromeric foci in the absence of HP1 During pericentromeric heterochromatin formation, HP1 is thought of as a crucial link between H3K9me3 and the stabilization of heterochromatinization mainly via recruitment of H4K20me3 and CpG methylation activity [5] . Eukaryotic cells have three HP1 isoforms, HP1α, HP1β and HP1γ, of which HP1α and HP1β localize preferentially to pericentromeric heterochromatin and have partially redundant functions [39] . To analyse H3K64me3 dependency on HP1, we made use of a double ko MEF line, deficient for both HP1α and HP1β isoforms (HP1α/β dko MEFs [40] ). Control immunofluorescence analyses demonstrated that both HP1 isoforms are absent in these mutant cells ( Supplementary Fig. S3a ). Analysis of H4K20me3 confirmed its dependency on HP1 at the pericentromeric heterochromatin [15] : whereas wt MEFs showed expected enrichment at heterochromatic foci, there was much reduced staining of DAPI-positive H4K20me3 foci in HP1 mutant cells ( Fig. 3a ). In contrast, pericentromeric heterochromatin enrichment of H3K9me3 was unaltered in mutant compared with control MEFs ( Fig. 3a [41] ). Next, we analysed H3K64me3 nuclear localization and global levels in HP1α/β dko cells. The observed staining pattern was comparable between wt and mutant cells, with pericentromeric heterochromatic foci readily detectable in cells deficient for HP1α and HP1β ( Fig. 3a ). Global levels of H3K64me3 were comparable to those of wt cells, similar to H3K9me3 levels ( Fig. 3b ; Supplementary Fig. S3b [41] ). In summary, these data demonstrate that HP1 is not required for the typical H3K64me3 enrichment at pericentromeric heterochromatin foci. 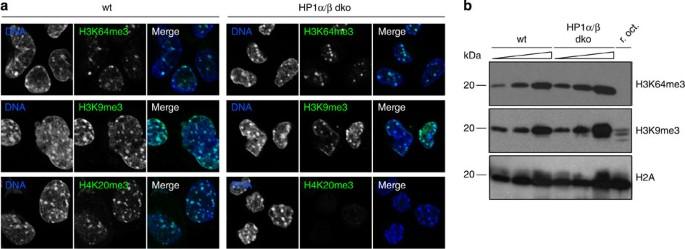Figure 3: Enrichment of H3K64me3 at PH foci is independent of HP1. (a) IF analysis of wt (left panels) and HP1α/β dko (right panels) MEFs using antibodies against H3K64me3, H3K9me3 and H4K20me3. DNA was counterstained with DAPI. Whereas H4K20me3 enrichment is lost at DAPI-intense heterochromatic foci in dko cells, the staining patterns for H3K64me3 and H3K9me3 are maintained. Scale bar, 10 μm. (b) Immunoblot analysis of native histones extracted from wt and HP1 dko MEFs shows no reduction in global H3K64me3 or H3K9me3 levels in dko cells. Increasing amounts of histones were loaded and a control with recombinant octamers is shown (r.oct.). Loading was controlled by blotting against H2A. Figure 3: Enrichment of H3K64me3 at PH foci is independent of HP1. ( a ) IF analysis of wt (left panels) and HP1α/β dko (right panels) MEFs using antibodies against H3K64me3, H3K9me3 and H4K20me3. DNA was counterstained with DAPI. Whereas H4K20me3 enrichment is lost at DAPI-intense heterochromatic foci in dko cells, the staining patterns for H3K64me3 and H3K9me3 are maintained. Scale bar, 10 μm. ( b ) Immunoblot analysis of native histones extracted from wt and HP1 dko MEFs shows no reduction in global H3K64me3 or H3K9me3 levels in dko cells. Increasing amounts of histones were loaded and a control with recombinant octamers is shown (r.oct.). Loading was controlled by blotting against H2A. Full size image Pericentromeric H3K64me3 foci are dependent on H3K9me3 We have shown previously that H3K64me3 at the pericentromeric heterochromatin is dependent on the presence of Suv39h protein, an H3K9-specific methyltransferase [10] . The nature of this dependency is, however, unclear and raises several questions. First, deposition of H3K64me3 could be mediated directly by Suv39h enzymatic activity. However, several histone methyltransferase assays using recombinant Suv39h enzymes with different substrates, including recombinant histones, octamers as well as native wt or H3K64-mutated nucleosomes, have refuted this possibility so far and have demonstrated no activity of Suv39h towards the H3K64 residue ( Fig. 4a , Supplementary Fig. S4a,b ). 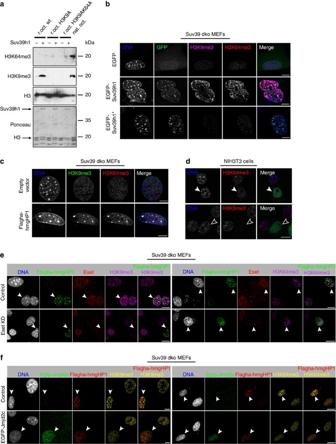Figure 4: H3K64me3 dependency on H3K9me3 at PH foci. (a)In vitromethylation assay using GST-tagged Suv39h1 methyltransferase on recombinant octamers containing wt H3, the H3K9A or H3K9AK64A mutant H3 as substrates. Subsequent immunoblot analysis using antibodies against H3K64me3 and H3K9me3 demonstrates the trimethylation activity of Suv39h1 on H3 for the K9 but not the K64 residue. Native octamers (nat. oct.) were used as positive control. (b) Suv39h1/h2 dko MEFs were transfected with wt EGFP-Suv39h1 and mutant, enzymatically inactive EGFP-Suv39h1* (green). IF stainings for H3K9me3 (purple) and H3K64me3 (red) show re-establishment of H3K9me3 and H3K64me3 at pericentromeric foci only in cells transfected with wt Suv39h1, although both wt EGFP-Suv39h1 and EGFP-Suv39h1* are able to localize to DAPI-dense foci. Scale bar, 10 μm. (c) Suv39h1/h2 dko MEFs were transfected with flagha-hmg.HP1 (lower panel) and an empty control vector (upper panel). Recruitment of HP1 to pericentromeric foci under the guidance of the AT-hook domain of hmgA1b results in H3K64me3 (red) restoration at PH foci in the absence of Suv39h1/h2 enzymes, as demonstrated using IF analysis. Note that H3K9me3 (green) enrichment at PH foci is also re-established in flagha-hmg.HP1-transfected cells. Scale bar, 10 μm. (d) NIH3T3 cells transfected with EGFP-tagged H3K9me3 demethylase Jmjd2c (arrows) lose pericentromeric foci enrichment of H3K64me3 and H3K9me3. Scale bar, 10 μm. (e) flagha-hmg.HP1-transfected Suv39h1/h2 dko MEFs were either subject to Eset/SetDB1 siRNA knockdown (Eset KD) or not (control). Eset/SetDB1 knockdown (Eset panels, red, white arrow) leads to the abolition of H3K9me3 (H3K9me3 panels, purple, white arrow) and H3K64me3 (H3K64me3 panels, purple, white arrow) restorations. (f) flagha-hmg.HP1-transfected Suv39h1/h2 dko MEFs were either transfected with EGFP-Jmjd2c (EGFP-Jmjd2c) or not (control). Concomitant expression of the EGFP-tagged H3K9me3 demethylase Jmjd2c (EGFP-Jmjd2c panels, green) prevents the restoration of H3K9me3 (H3K9me3 panels, yellow) and H3K64me3 (H3K64me3 panels, yellow). Scale bar, 20 μm. In (b–f) DNA was counterstained with DAPI. Figure 4: H3K64me3 dependency on H3K9me3 at PH foci. ( a ) In vitro methylation assay using GST-tagged Suv39h1 methyltransferase on recombinant octamers containing wt H3, the H3K9A or H3K9AK64A mutant H3 as substrates. Subsequent immunoblot analysis using antibodies against H3K64me3 and H3K9me3 demonstrates the trimethylation activity of Suv39h1 on H3 for the K9 but not the K64 residue. Native octamers (nat. oct.) were used as positive control. ( b ) Suv39h1/h2 dko MEFs were transfected with wt EGFP-Suv39h1 and mutant, enzymatically inactive EGFP-Suv39h1* (green). IF stainings for H3K9me3 (purple) and H3K64me3 (red) show re-establishment of H3K9me3 and H3K64me3 at pericentromeric foci only in cells transfected with wt Suv39h1, although both wt EGFP-Suv39h1 and EGFP-Suv39h1* are able to localize to DAPI-dense foci. Scale bar, 10 μm. ( c ) Suv39h1/h2 dko MEFs were transfected with flagha-hmg.HP1 (lower panel) and an empty control vector (upper panel). Recruitment of HP1 to pericentromeric foci under the guidance of the AT-hook domain of hmgA1b results in H3K64me3 (red) restoration at PH foci in the absence of Suv39h1/h2 enzymes, as demonstrated using IF analysis. Note that H3K9me3 (green) enrichment at PH foci is also re-established in flagha-hmg.HP1-transfected cells. Scale bar, 10 μm. ( d ) NIH3T3 cells transfected with EGFP-tagged H3K9me3 demethylase Jmjd2c (arrows) lose pericentromeric foci enrichment of H3K64me3 and H3K9me3. Scale bar, 10 μm. ( e ) flagha-hmg.HP1-transfected Suv39h1/h2 dko MEFs were either subject to Eset/SetDB1 siRNA knockdown (Eset KD) or not (control). Eset/SetDB1 knockdown (Eset panels, red, white arrow) leads to the abolition of H3K9me3 (H3K9me3 panels, purple, white arrow) and H3K64me3 (H3K64me3 panels, purple, white arrow) restorations. ( f ) flagha-hmg.HP1-transfected Suv39h1/h2 dko MEFs were either transfected with EGFP-Jmjd2c (EGFP-Jmjd2c) or not (control). Concomitant expression of the EGFP-tagged H3K9me3 demethylase Jmjd2c (EGFP-Jmjd2c panels, green) prevents the restoration of H3K9me3 (H3K9me3 panels, yellow) and H3K64me3 (H3K64me3 panels, yellow). Scale bar, 20 μm. In ( b – f ) DNA was counterstained with DAPI. Full size image Second, the presence of Suv39h protein could be required as a structural component in order to recruit H3K64me3 activity towards constitutive heterochromatin. To test this possibility, we transiently transfected Suv39h1/h2 double ko mutant cells (dko) with EGFP-tagged wt Suv39h1 or enzymatic-dead Suv39h1H324K [18] and assayed for restoration of H3K64me3 levels at the pericentromeric heterochromatic foci. Figure 4b demonstrates that, whereas Suv39h wt is able to restore both H3K9me3 and H3K64me3 at pericentromeric heterochromatic foci, the enzymatic-dead mutant is incapable despite its localization to these regions. These observations indicate that Suv39h protein as a structural component is insufficient for recruiting H3K64me3 activity. To obtain further insight into the mechanism and interplay between H3K64me3 and H3K9me3, we investigated a potential dependency of H3K64me3 on H3K9me3 at pericentromeric heterochromatin in an experimental setup, in which H3K9me3 is artificially recruited to pericentromeric heterochromatin in Suv39h1/h2 dko cells. This restoration of pericentromeric H3K9me3 foci is possible by the targeting of HP1 to pericentromeric heterochromatin under guidance of the AT-hook domains of hmgA1b that binds to AT-rich pericentromeric heterochromatin ( Supplementary Fig. S4c [42] ). In the absence of Suv39h1/h2, the H3K9 methyltransferase Eset/SetDB1 is recruited through hmg.HP1 [42] and ectopically restores H3K9me3 at pericentromeric heterochromatin ( Fig. 4c ). Importantly, we find that restoring H3K9me3 at the pericentromeric heterochromatin foci in this context can lead to concomitant restoration of H3K64me3 at these sites ( Fig. 4c ). This suggests that H3K64me3 enrichment at pericentromeric heterochromatin foci can occur independent of Suv39h, but requires the presence of H3K9me3. In support of this observation, removal of the H3K9me3 marker by transiently expressing H3K9me3 demethylases Jmjd2c and Jmjd2d in NIH3T3 cells [43] , [44] , [45] also leads to marked reduction in H3K64me3 enrichment at the pericentromeric foci ( Fig. 4d ; Supplementary Fig. S4d ). Notably, a histone demethylase bearing specificity towards a different residue fails to influence H3K64me3 or H3K9me3 levels ( Supplementary Fig. S4d ). To further corroborate these results, we also prevented the restoration of H3K9me3 at pericentromeric heterochromatin in hmg.HP1-expressing Suv39h1/h2 dko cells through the depletion of Eset/SetDB1 by short interfering RNA (siRNA) knockdown ( Fig. 4e ) or overexpression of Jmjd2c ( Fig. 4f ). In both circumstances, H3K64me3 restoration at the pericentromeric heterochromatin foci is abolished ( Fig. 4e,f ). Together, our findings strongly suggest that H3K64me3 deposition at the foci of pericentromeric heterochromatin is H3K9me3-dependent, providing a functional link between these two hallmarks of pericentromeric heterochromatin. H3K64me3 supports pericentromeric heterochromatin integrity To investigate a possible functional impact of H3K64me3 on the integrity of pericentromeric heterochromatin, we next aimed to manipulate H3K64me3 levels. To date, no specific enzymatic activity for trimethylation of H3K64 has been identified. We therefore made use of the expression of wt H3 and an H3K64 to the R mutant (not methylatable), targeted to pericentromeric heterochromatin via hmg-AT-hook domains [42] . This approach allowed us to test for a possible impact of manipulation of H3K64 modification levels on pericentromeric heterochromatin integrity. Interestingly, we observed that expression of the H3K64R mutant can act in a dominant-negative manner, and, compared with the expression of the hmg-AT/hook alone ( Supplementary Fig. S5a ) or a wild-type hmg.H3 fusion ( Supplementary Fig. S5b ), hmg.H3K64R can lead to alterations in pericentromeric heterochromatin ( Supplementary Fig. S5c ). Expression of non-methylatable H3K64R seems to markedly impair normal enrichment of the hallmarks of constitutive heterochromatin, namely, H3K9me3 ( Fig. 5a , Supplementary Fig. S5c ), HP1 and H4K20me3 ( Fig. 5b , Supplementary Fig. S5c ), at pericentromeric heterochromatin foci in mouse NIH3T3 cells. These data imply a reverse relationship of dependency of known pericentromeric heterochromatin markers on H3K64me3 and suggest a key role for H3K64me3 in reinforcing heterochromatic integrity at the pericentromere. 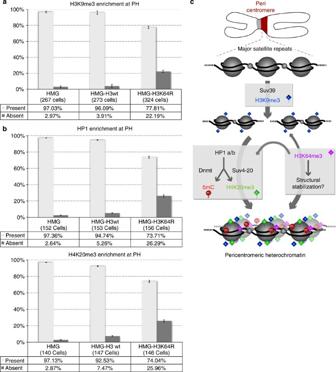Figure 5: H3K64me3 is important for maintaining PH integrity. (a) NIH3T3 cells transfected with K64-non-methylatable flagha-hmg.H3K64R mutant show (compared with flagha-hmg.H3 wild-type (wt) transfected cells) impaired PH integrity as revealed by perturbed enrichment of the heterochromatin hallmark H3K9me3. Graph shows the percentage of cells displaying normal enrichment (grey bars: present) or absence (black bars: absent) of this hallmark of heterochromatin after transfection and specific expression of fagha-hmg, flagha-hmgH3 wt or flagha-hmgH3K64R mutant at PH. Means of two replicates from two independent experiments are represented. Error bars represent range. (b) The same transfection experiment shows impaired PH integrity as revealed by perturbed enrichment of two H3K9me3-dependent heterochromatin hallmarks, HP1 (upper graph) and H4K20me3 (lower graph). Means of two independent experiments are represented. Error bars represent range. Note that only the flagha-hmgH3K64R mutant markedly compromises heterochromatin integrity, leading to an increase of, in certain cases, over 20% of cells, in which hallmarks disappeared from PH foci.(c) Model of heterochromatinization events at the pericentromere. Suv39 enzymes are targeted by a yet unknown mechanism to repeat-rich pericentromeric chromatin, resulting in enrichment of H3K9me3. Consequently, chromatin binding and modifying enzymes are recruited to these regions, involving HP1 proteins and, downstream thereof, Dnmts and Suv4-20 enzymes. H3K9me3 also promotes H3K64me3 deposition, leading potentially to structural stabilization of chromatin by strengthening DNA–histone octamer interactions. H3K64me3 itself could furthermore reinforce heterochromatin integrity by locally stabilizing H3K9me3, HP1 and H4K20me3. Thus, trimethylation of H3 at K64 seems important for the formation of a robust heterochromatin at pericentromeric sites, characterized by high levels of H3K9me3, H3K64me3, CpG methylation and H4K20me3. See text for details. Figure 5: H3K64me3 is important for maintaining PH integrity. ( a ) NIH3T3 cells transfected with K64-non-methylatable flagha-hmg.H3K64R mutant show (compared with flagha-hmg.H3 wild-type (wt) transfected cells) impaired PH integrity as revealed by perturbed enrichment of the heterochromatin hallmark H3K9me3. Graph shows the percentage of cells displaying normal enrichment (grey bars: present) or absence (black bars: absent) of this hallmark of heterochromatin after transfection and specific expression of fagha-hmg, flagha-hmgH3 wt or flagha-hmgH3K64R mutant at PH. Means of two replicates from two independent experiments are represented. Error bars represent range. ( b ) The same transfection experiment shows impaired PH integrity as revealed by perturbed enrichment of two H3K9me3-dependent heterochromatin hallmarks, HP1 (upper graph) and H4K20me3 (lower graph). Means of two independent experiments are represented. Error bars represent range. Note that only the flagha-hmgH3K64R mutant markedly compromises heterochromatin integrity, leading to an increase of, in certain cases, over 20% of cells, in which hallmarks disappeared from PH foci. ( c ) Model of heterochromatinization events at the pericentromere. Suv39 enzymes are targeted by a yet unknown mechanism to repeat-rich pericentromeric chromatin, resulting in enrichment of H3K9me3. Consequently, chromatin binding and modifying enzymes are recruited to these regions, involving HP1 proteins and, downstream thereof, Dnmts and Suv4-20 enzymes. H3K9me3 also promotes H3K64me3 deposition, leading potentially to structural stabilization of chromatin by strengthening DNA–histone octamer interactions. H3K64me3 itself could furthermore reinforce heterochromatin integrity by locally stabilizing H3K9me3, HP1 and H4K20me3. Thus, trimethylation of H3 at K64 seems important for the formation of a robust heterochromatin at pericentromeric sites, characterized by high levels of H3K9me3, H3K64me3, CpG methylation and H4K20me3. See text for details. Full size image Constitutive heterochromatin at the pericentromere carries a specific signature of chromatin modifications. Targeted deposition of H3K9me3 by Suv39 enzymes is thought to be one of the most upstream events, leading to the recruitment of HP1. This central factor not only directs Suv4-20 enzymes and their H4K20me3 product to constitutive heterochromatin but also brings about DNA methyltransferases, methyl-CpG-binding proteins and histone deacetylases [11] . This cascade of events is proposed to stabilize constitutive heterochromatin. Here we integrate for the first time the histone core domain trimethylation of H3K64 in this pathway. On the basis of our findings, we propose a model in which H3K64me3 helps to stabilize pericentromeric heterochromatin in an H3K9me3-dependent manner and participates in a self-reinforcing feedback loop to ensure heterochromatic integrity ( Fig. 5c ). Interestingly, our results indicate no dependence of H3K64me3 on DNA methylation or H4K20me3, two well-characterized factors of constitutive heterochromatin formation. Notably, H3K64me3 placement at the pericentromeric heterochromatin foci is also independent of the central heterochromatic component HP1. This importantly sets H3K64me3 apart from the known pathway of heterochromatinization at the pericentromere and also raises the possibility of a potential H3K64me3-binding protein. Such a specific reader could argue for a heterochromatinization cascade complementary to the pathway involving HP1-mediated recruitment. So far, we have been unable to identify such a specific H3K64me3 binder. It is conceivable that the particular localization of H3K64me3 at the lateral surface of the histone octamer impedes access for potential binding proteins, and H3K64me3 marking in repressive chromatin might alternatively fulfil a structural role [10] , [46] , [47] , [48] . We find the repressive hallmark H3K9me3 to be key for H3K64me3 targeting. This observed dependency appears to be directly linked to the presence of H3K9me3, rather than to H3K9-methylating enzyme Suv39. It raises the question whether a yet unidentified enzymatic activity responsible for H3K64me3 catalysis may be targeted to constitutive heterochromatin through binding to H3K9me3 and/or dependent on H3K9me3-enriched environments—for example, via an H3K9me3-binding protein other than HP1. As far as the removal of H3K64me3 is concerned, we show that two H3K9me3 demethylases are capable of antagonizing H3K64me3. Whether these demethylases act on H3K64me3 or whether the observed loss is secondary to reduction in H3K9me3 levels needs further investigation, especially as previous reports have demonstrated that several histone demethylases are capable of acting on more than one residue, in particular when methylation of these residues is associated with a similar functional chromatin state [49] , [50] . Our data finally draw attention to several intriguing aspects concerning the causal interplay of H3K64me3 and other pericentromeric heterochromatin markers. Although we see no dependency of H3K64me3 on DNA methylation, H4K20me3 and HP1, our data suggest that the reverse might be the case. In fact, reinforcing feedback loops during heterochromatinization of pericentromeric regions have previously been reported, with HP1 interacting with Suv39h1/h2 enzymes to amplify H3K9me3 marking [11] , [22] . In line with this, our results show that expressing an H3K64R mutant can severely compromise heterochromatin integrity. These data suggest a novel feedback loop involving H3K64me3 and H3K9me3, whereby H3K64me3 would reinforce heterochromatinization by promoting recruitment and/or maintenance of key heterochromatic factors such as HP1 or H3K9me3 ( Fig. 5c ). In conclusion, we hypothesize that H3K64me3 at pericentromeric repeats accounts for a key mechanism to ensure heterochromatin integrity. Once chromatin at the pericentromere has been methylated at H3K9, two mechanisms would ensure robust heterochromatinization at these sites: first, H3K9me3-dependent recruitment of non-histone proteins and chromatin modifiers, warranting the establishment of a repressive chromatin signature; second, stabilization of DNA–histone octamer interactions by methylation of H3K64, a residue at the lateral surface of the histone octamer. H3K64me3 could further reinforce local heterochromatinization by positively having an impact on H3K9me3 and HP1 ( Fig. 5c ). In this way a stable heterochromatic environment could be formed, crucially ensuring genomic stability. In the future, it will be exciting to dissect the distinct roles and complementary impact of H3K64me3 and H3K9me3 on heterochromatin function in further detail. Cell culture and transfection assays Cell lines were kind gifts from M. Muto (NP95 ko ES cells; E14 wt ES cells), M. Okano (Dnmt1/3a/3b ES cells; J1 wt ES cells), P. Singh (HP1a/b dko MEFs; wt MEFs) and T. Jenuwein (Suv4-20h1/h2 dko MEFs; Suv39h1/h2 dko MEFs; wt MEFs). ES and MEF cell lines were cultivated in DMEM (PAA) supplemented with 10% (15% for ES cells) fetal calf serum (Perbio), high glucose (4.5 g l −1 ), L -glutamine (2 mM, PAA), sodium pyruvate (1 mM, Millipore), non-essential amino acids (1X, Sigma-Aldrich), Beta-mercaptoethanol (100 μM, Millipore), penicillin/streptomycin (1X, PAA) and Leukemia inhibitory factor (LIF) for ES cells. Cells were grown at 37 °C in an atmosphere of 5% CO 2 and maximum humidity [14] . Transfection assays were carried out using Fugene HD and X-tremeGENE HD reagents (Roche) according to the manufacturer’s instructions, and cells were analysed 48–72 h post transfection. Expression constructs were generated using conventional or Gateway cloning systems (Invitrogen). Gateway entry clones containing mouse JmjC-domain cDNAs were kindly donated by R. Schuele. A domain containing the three AT hooks (amino acids 1–81) of the mouse hmgA1b was PCR-amplified from NIH3T3 cells and subcloned between the N-terminal flag-2ha tags and mouse HP1α cDNA in the mammalian expression vector pcDNA3.1. This construct allows artificial recruitment to mouse pericentromeric heterochromatin by targeting fusion proteins to pericentromeric heterochromatin under the guidance of AT-hook domains of hmgA1b that bind to AT-rich pericentromeric heterochromatin [42] . Using this flagha-hmg.HP1 construct, a flagha-hmg-expressing vector was created. PCR-amplified wild-type human histone H3 (H3wt) was inserted into the flagha-hmg vector in order to artificially target the flagha-hmg-H3wt fusion specifically to pericentromeric heterochromatin foci. The K64 to R mutation of H3 was created in the same vector backbone to target a K64-non-methylatable flagha-hmg.H3K64R mutant to pericentromeric heterochromatin foci. The EGFP-Suv39h1 mammalian expression vector was a gift from C. Galan and T. Jenuwein. The catalytic dead mutant was constructed in the same backbone by mutating histidine 324 to Lysine (EGFP-Suv39h1-H324K), which has been shown to completely inactivate the Suv39h1 histone methyltransferase activity [18] . Testing for the abolition of H3K9me3 and H3K64me3 restoration in flagha-hmg.HP1-transfected Suv39 dko MEFs was achieved using two approaches: Eset/SetDB1 knockdown in Suv39 dko MEFs was carried out by transfecting specific SMARTpool siRNA (Dharmacon, M-040815-01-0005) concomitantly with flagha-hmg.HP1-expressing vector using DharmaFECT Duo reagent for siRNA and plasmid cotransfection (Dharmacon). The second approach involved cotransfection of flagha-hmg.HP1 and EGFP-Jmjd2c-expressing vectors into Suv39 dko MEFs using X-tremeGENE HD reagents (Roche). Cell cycle synchronization and analysis Human T24 cells were used for their ability to be synchronized by letting them grow to confluency without the need for more drastic methods such as double thymidine block. Keeping cells at 100% confluency for 5 days leads to arrest in the G0 state. To re-enter the cell cycle, cells were diluted in a new plate and collected for flow cytometry or histone extraction and western blotting analysis after appropriate periods of time. Cell cycle distribution was checked by propidium iodide staining and fluorescent activated cell sorting (FACS) as described by Darzynkiewicz et al. [51] Histones from the different cell cycle stages were extracted in parallel as described in this manuscript and analysed using western blotting with secondary antibodies coupled to fluorophores to quantify signal with an Odyssey Infrared Imaging System (LI-COR Biosciences). Embryo collection and Tet knockdown experiments All animal experiments were carried out according to the German Animal Welfare law in agreement with the authorizing committee. Briefly, for the knockdown experiments, siRNAs (2 μM each) were co-injected with Dextran-tetramethyl-rhodamine (Invitrogen, 3,000 MW, 100 μg ml −1 ) into MII-arrested oocytes derived from superovulated F1(C57BL/6 × DBA) mice according to Wossidlo et al. [37] After 8 h of incubation at 37 °C in a humidified atmosphere of 5% CO 2 and 95% air, siRNA-injected oocytes were fertilized by intracytoplasmic sperm injection with capacitated sperm derived from F1(C57BL/6 × DBA) mice. After 7 h of cultivation, G1-phase zygotes were collected in M2 medium and the zona pellucida was removed by treatment with acidic tyrodes solution. Subsequently, the zygotes were fixed for 20 min in 3.7% paraformaldehyde in PBS at 4 °C and permeabilized with 0.2% Triton X-100 in PBS for 10 min at room temperature (RT). The fixed zygotes were blocked overnight at 4 °C in 1% bovine serum albumin (BSA) 0.1% Triton X-100 in PBS. Next, fixed zygotes were analysed for 5mC, 5hmC and H3K64me3 by immunostaining as described below. The 5′ to 3′ sense sequences of siRNA [37] were Tet1: 5′-AAGAAGCAGTGTACACATAAT-3′ and 5′-GCAGATGGCCGTGACACAAAT-3′; Tet2: 5′-AAGGCCTGTGATGCTGATAAT-3′ and 5′-GGATGTAAGTTTGCCAGAAGC-3′; Tet3: 5′-AAGCGCAACCTATTCTTGGAA-3′; and scramble: 5′-GCCTGAGCGATTATAACCTTT-3′ Immunofluorescence stainings Cells were plated onto gelatin-coated coverslips (MEFs, NIH3T3) or cytospin-fixed after trypsinization onto histology slides (ES cell lines). Cells were fixed in PBS, 4% PFA and 2% sucrose for 10 min at RT and washed 4 × in PBS before permeabilization in PBS and 0.6% Triton X-100, for 20 min at RT. Cells were then blocked in PBS, 4% BSA and 0.2% Tween-20 for 1 h at RT and antibody staining was carried out in the same buffer at 4 °C overnight with an H3K64me3-specific antibody (used at 1/250), generated, affinity-purified and tested for cross-reactivity as previously described [10] . Additional antibodies including anti-H3K9me3 (mouse monoclonal (1/250)), Active Motif and rabbit polyclonal ((1/400) Millipore), anti-H4K20me3 ((1/250) Millipore), anti-MeCP2 ((1/200) Cell Signalling Technology), anti-HP1α ((1/200) Upstate), anti-HP1β ((1/100) Abcam), anti-NP95 ((1/200) kind gift from I. Bonapace), anti-Eset ((1/75) Santa Cruz), anti-HA(1/600) and anti-Flag (1/300) were also used for stainings. The coverslips were subsequently washed 3 × in PBS and 4% BSA, and incubated with fluorochrome-conjugated secondary antibodies (anti-mouse, anti-rabbit or anti-goat conjugated to Rhodamine Red-X, Alexa Fluor 488 or Alexa Fluor 647 (3 μg ml −1 ) Jackson ImmunoResearch) for 1 h at RT in the dark, washed 3 × in PBS, 4% BSA and 1 × in PBS. The coverslips were then mounted in Vectashield with DAPI (Vector laboratories). For the anti-5mC (Calbiochem) and anti-5hmC (Active Motif) immunostaining studies, fixed zygotes were incubated in 4 N HCl solution at RT for 15 min. Following neutralization (10 min 100 mM Tris-HCl, pH 8.0) and second fixation, the embryos were stained with anti-5hmC (rabbit polyclonal (1:100)) and anti-5mC (mouse monoclonal (1:2,000)). After several washes in blocking solution, the embryos were incubated at RT with anti-mouse secondary antibodies for 2 h coupled with Alexa Fluor 488 (10 μg ml −1 ) and anti-rabbit secondary antibodies coupled with Rhodamine Red-X (15 μg ml −1 , Jackson ImmunoResearch Laboratories). Zygotes were then washed and mounted on slides in Vectashield with DAPI. Confocal imaging was carried out using either a Leica SP2, a Zeiss LSM680 or a Zeiss Axiovert 200 M inverted microscope. Histone extraction and western blot analysis To prepare native histones, nuclei were isolated from cells by incubating them for 10 min in TEB buffer (0.5% Triton X-100 in PBS) and then acid-extracted with 0.2 N HCl for 3–4 h at 4 °C. After extraction, protein concentration was determined and equal amounts of protein were separated on SDS–PAGE and transferred onto nitrocellulose membrane before conventional western blotting experiments using anti-H3K9me3 (mouse monoclonal (1/1,000)), Active Motif and rabbit polyclonal (1/2,000) Millipore), anti-H3K64me3 (1/2,000), anti-H3 ((1/10,000) Abcam) and anti-H2A ((1/3,000) Millipore). In vitro histone methyltransferase assay Briefly, 1 μg of purified recombinant human octamers containing either wild-type or mutated H3 (K9A or K9AK64A) [52] were mixed with 1 μg of purified recombinant GST-Suv39h1 and incubated in methylation buffer (50 mM Tris-HCl, pH 8.5, 20 mM KCl, 10 mM MgCl 2 , 0.25 mM sucrose) containing 5 μM S -adenosyl-methionine (SAM) as methyl donor at 30 °C for 90 min [18] . Histone methyltransferase reactions were stopped by boiling in SDS-loading buffer, and proteins were separated using 18.7% SDS–PAGE before being transferred onto nitrocellulose and immunoblotted as described in the Histone extraction and western blot analysis section. How to cite this article: Lange U. C. et al. Dissecting the role of H3K64me3 in mouse pericentromeric heterochromatin. Nat. Commun. 4:2233 doi: 10.1038/ncomms3233 (2013).